DNMT1 is essential for mammary and cancer stem cell maintenance and tumorigenesis Mammary stem/progenitor cells (MaSCs) maintain self-renewal of the mammary epithelium during puberty and pregnancy. DNA methylation provides a potential epigenetic mechanism for maintaining cellular memory during self-renewal. Although DNA methyltransferases (DNMTs) are dispensable for embryonic stem cell maintenance, their role in maintaining MaSCs and cancer stem cells (CSCs) in constantly replenishing mammary epithelium is unclear. Here we show that DNMT1 is indispensable for MaSC maintenance. Furthermore, we find that DNMT1 expression is elevated in mammary tumours, and mammary gland-specific DNMT1 deletion protects mice from mammary tumorigenesis by limiting the CSC pool. Through genome-scale methylation studies, we identify ISL1 as a direct DNMT1 target, hypermethylated and downregulated in mammary tumours and CSCs. DNMT inhibition or ISL1 expression in breast cancer cells limits CSC population. Altogether, our studies uncover an essential role for DNMT1 in MaSC and CSC maintenance and identify DNMT1-ISL1 axis as a potential therapeutic target for breast cancer treatment. Mammary epithelium undergoes multiple rounds of proliferation, differentiation and apoptosis during pregnancy, lactation and involution [1] , [2] . Classical transplantation assays, lineage tracing and cell-fate mapping studies in mice have revealed the existence of a hierarchy of stem and progenitor cells among the mammary epithelium [3] , [4] , with a considerable increase in mammary stem cell (MaSC) activity during pregnancy [5] . Given the increased risk of breast cancer associated with pregnancy in the short term, the augmented MaSC pool has been postulated to be the cellular basis for increased breast cancer incidence during pregnancy [5] . The maintenance of stem/progenitor cells and their differentiation fate in the mammary epithelium follows a well-defined epigenetic programme, with a growing number of chromatin regulators implicated in controlling the homeostatic balance between self-renewal and differentiation state [6] , [7] . DNA methylation is among the best-studied epigenetic modification [8] , which provides a potential mechanism for maintaining cellular memory during repeated cell divisions [9] . Embryonic stem cells (ESCs) that lack DNA methyltransferases (DNMTs) are viable, but die when induced to differentiate [10] , [11] , [12] , suggesting that proper establishment and maintenance of DNA methylation patterns are essential for mammalian development and for the normal functioning of the adult organism [13] . Indeed, a growing number of human diseases including cancer have been found to be associated with aberrant DNA hypermethylation at CpG islands, most of which are unmethylated in normal somatic cells [13] . As de novo methylation of CpG islands is widespread in tumour cells and is an early event in transformation [14] , [15] , it represents an excellent biomarker for early cancer detection [16] . Dnmt1 is essential for the maintenance of haematopoietic stem cells (HSCs)/progenitor cells [17] , epidermal progenitor cells [18] , mesenchymal stem cells [19] and leukemia stem cells [20] , but its role in the regulation of mammary stem/progenitor cells and mammary tumorigenesis has not been studied. Here we show that Dnmt1 is required for mammary gland outgrowth and terminal end bud (TEB) development, and that mammary-gland-specific Dnmt1 deletion in mice leads to significant reduction in mammary stem/progenitor cells. We also show that Dnmt1 deletion or inhibition of Dnmt1 activity almost completely abolishes Neu-Tg- and C3(1)-SV40-Tg-driven mammary tumour formation and metastasis, a phenomenon that is associated with significant reduction in cancer stem cells (CSCs). Through genome-scale DNA methylation studies in normal and CSCs, we find ISL1 , an endogenous inhibitor of oestrogen receptor (ER)-driven transcription activation [21] , is hypermethylated in CSCs and silenced in most human breast cancers. Functional re-expression of ISL1 or inhibition of DNMT activity in breast cancer cells reduces cell growth, migration and CSC formation. Our studies provide the first in-vivo evidence showing a requirement for DNMT1 in mammary stem/progenitor cell and CSC maintenance, and identify DNMT1-ISL1 axis as a potential therapeutic target for breast cancer treatment. Dnmt1 expression during mammary gland development We investigated Dnmt1 expression during different stages of mammary gland development and observed significantly higher levels of Dnmt1 expression in mid-pregnant mammary gland ( Fig. 1a–c ) along with a dramatic increase in stem cell-enriched basal cells (Lin − CD49f high CD24 + ) and luminal cells (Lin − CD49f low CD24 + ) ( Fig. 1d,e ). Isolation of Lin − CD49f high CD24 + and Lin − CD49f low CD24 + cells from 8-week-old virgin mammary glands revealed that both cell populations expressed similar levels of Dnmt1 ( Supplementary Fig. 1a–c ). To determine the role of Dnmt1 in the regulation of mammary stem/progenitor cells, we generated mammary gland-specific conditional Dnmt1 -knockout mice, as global deletion of Dnmt1 leads to early embryonic lethality [11] . We bred mice in which loxP sites flanked exons 4 and 5 of the Dnmt1 gene [11] , with mice expressing Cre recombinase under the control of MMTV promoter. Dnmt1 deletion in the mammary gland was confirmed by the loss of Dnmt1 expression and significant reduction in DNA methylation levels ( Supplementary Fig. 1d–h ). To evaluate Dnmt1’s role in mammary epithelium, we analysed mammary glands from wild-type ( Dnmt1 fl/fl ) and Dnmt1- knockout ( Dnmt1 Δ/Δ ) female littermates by whole-mount analysis. At 7 weeks post partum, mammary ducts colonize ∼ 55%–60% of the fat pad in Dnmt1 fl/fl mice, and TEBs that contain stem cells and their highly proliferative progeny extend beyond the lymph nodes ( Fig. 1f,g ). In contrast, the development of the mammary gland in Dnmt1 Δ/Δ littermates was severely inhibited. In the mammary gland, a subpopulation of cells located in the basal layer of terminal end ducts has been implicated as stem cells. We found that deletion of Dnmt1 severely affected TEB development in the virgin mammary glands ( Fig. 1h,i ). 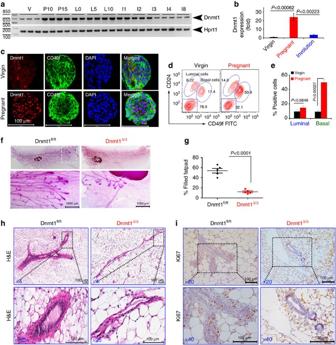Figure 1: Dnmt1 expression during mammary gland development (a)Dnmt1gene transcript levels were analysed in the mammary glands harvested from virgin (V), pregnant days 10 and 15 (P10 and P15), lactation days 0, 5 and 10 (L0, L5 and L10), and involution days 1, 2, 3, 4 and 8 (I1, I2, I3, I4 and I8) mice. Hprt1 was used as a loading control. (n=3 mice in each time point). (b) Real-time PCR showing relative expression ofDnmt1from virgin, pregnancy and involution stage (n=3). (c) Representative immunofluorescence (IF) staining for Dnmt1 (red), CD49f (green) and DAPI (4′-6-diamidino-2-phenylindole; blue) in mammospheres generated with cells from virgin mice and pregnant mice at 10th day of gestation (n=3). Scale bar, 100 μm. (d) Representative contour plots of FACS gating showing a fourfold increase in basal myoepithelial stem cells in mammary glands of pregnant mice at 10th day of gestation compared with mammary glands of virgin mice (n=3–5). (e) Bar diagram showing per cent positive basal and luminal cells in virgin and pregnant mice. Data represents mean±s.d. of four independent mice in each group. (f) Carmine staining of inguinal mammary glands from 7-week-old wild-type (Dnmt1fl/fl) andDnmt1-knockout (Dnmt1Δ/Δ) littermates shows severe delay in TEB development inDnmt1-knockout mice (n=3). LN, for lymph node. Scale bar, 100 μm. (g) Quantification for per cent fat pad filled in the mammary gland (n=3). (h) Haematoxylin and eosin (H&E)-stained image of wild-type andDnmt1Δ/Δmouse mammary gland sections show severe defect in mammary gland development. Images were taken at × 4 and × 20 magnifications (n=3). Scale bar, 100 μm. (i) Ki67-stained section and histogram of wild-type andDnmt1Δ/Δmammary glands show significantly reduced Ki67 staining inDnmt1Δ/Δmice. Images were taken at × 20 and × 40 magnifications. Scale bar, 100 μm. Statistical analysis was performed using unpaired Student’st-tests. Error bars represent s.e.m. of independent experiments. Figure 1: Dnmt1 expression during mammary gland development ( a ) Dnmt1 gene transcript levels were analysed in the mammary glands harvested from virgin (V), pregnant days 10 and 15 (P10 and P15), lactation days 0, 5 and 10 (L0, L5 and L10), and involution days 1, 2, 3, 4 and 8 (I1, I2, I3, I4 and I8) mice. Hprt1 was used as a loading control. ( n =3 mice in each time point). ( b ) Real-time PCR showing relative expression of Dnmt1 from virgin, pregnancy and involution stage ( n =3). ( c ) Representative immunofluorescence (IF) staining for Dnmt1 (red), CD49f (green) and DAPI (4′-6-diamidino-2-phenylindole; blue) in mammospheres generated with cells from virgin mice and pregnant mice at 10th day of gestation ( n =3). Scale bar, 100 μm. ( d ) Representative contour plots of FACS gating showing a fourfold increase in basal myoepithelial stem cells in mammary glands of pregnant mice at 10th day of gestation compared with mammary glands of virgin mice ( n =3–5). ( e ) Bar diagram showing per cent positive basal and luminal cells in virgin and pregnant mice. Data represents mean±s.d. of four independent mice in each group. ( f ) Carmine staining of inguinal mammary glands from 7-week-old wild-type ( Dnmt1 fl/fl ) and Dnmt1 -knockout ( Dnmt1 Δ/Δ ) littermates shows severe delay in TEB development in Dnmt1 -knockout mice ( n =3). LN, for lymph node. Scale bar, 100 μm. ( g ) Quantification for per cent fat pad filled in the mammary gland ( n =3). ( h ) Haematoxylin and eosin (H&E)-stained image of wild-type and Dnmt1 Δ/Δ mouse mammary gland sections show severe defect in mammary gland development. Images were taken at × 4 and × 20 magnifications ( n =3). Scale bar, 100 μm. ( i ) Ki67-stained section and histogram of wild-type and Dnmt1 Δ/Δ mammary glands show significantly reduced Ki67 staining in Dnmt1 Δ/Δ mice. Images were taken at × 20 and × 40 magnifications. Scale bar, 100 μm. Statistical analysis was performed using unpaired Student’s t -tests. Error bars represent s.e.m. of independent experiments. Full size image Dnmt1 is indispensable for MaSC maintenance To understand the role of Dnmt1 in the development of mammary gland cellular lineages, we prepared single-cell suspensions from mammary glands isolated from Dnmt1 fl/fl and Dnmt1 Δ/Δ female mice. Flow cytometry analysis showed that Dnmt1 deletion decreased MaSC-enriched basal cells (Lin − CD49f high CD24 + ) and luminal cells (Lin − CD49f low CD24 + ) ( Fig. 2a ). Further analysis of the luminal cells using the CD61 marker, which distinguishes between luminal progenitor (LP) cells (Lin − CD49f low CD61 + , ER negative) and mature luminal cells (Lin − CD49f low CD61 − , ER positive), revealed a significant decrease in LPs ( Fig. 2b ). This decrease in MaSCs and progenitor cells is consistent with low mammosphere formation ( Fig. 2c ) and Ki67 expression ( Fig. 1i ), and low frequency of mammary repopulating unit in Dnmt1 Δ/Δ mice compared with Dnmt1 fl/fl mice ( Supplementary Fig. 2 ). Together, these observations show that Dnmt1 plays a key role in mammary gland development, and that deletion of Dnmt1 severely disrupts TEB development that grows out from MaSCs. 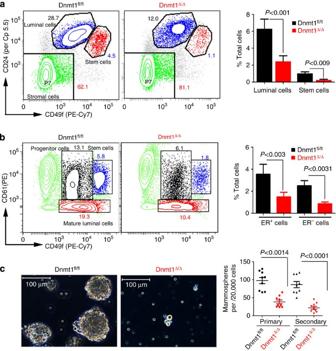Figure 2: Dnmt1 is indispensable for mammary stem/progenitor cell maintenance. (a) Single-cell suspensions from mammary glands of Dnmt1fl/fland Dnmt1Δ/Δmice were stained with CD24, CD49f and Lin (CD31, CD45 and CD119) antibodies. Representative FACS dot blots showing reduced stem (Lin−CD49fhighCD24+) and luminal cells (Lin−CD49flowCD24+) inDnmt1-knockout mice (n=3–5 mice in each). Bar diagram represents per cent of total stem and luminal cell populations in the respective mammary glands. (b) Similarly, single-cell suspensions from mammary glands ofDnmt1fl/flandDnmt1Δ/Δmice were stained with CD61, CD49f and Lin antibodies. Representative contour blots show reduced luminal progenitor cells (Lin−CD49flowCD61+) inDnmt1-knockout mice. Bar diagram represents per cent of total ER+and ER−cell populations in the respective mammary glands. (c) Representative images show a decrease in size and number in mammospheres generated with cells fromDnmt1Δ/Δmice compared with cells from Dnmt1fl/flmice (n=3–5). Twenty thousand cells per ml were used in each group. Bar diagram represents total number of mammospheres per 20,000 cells. Scale bar, 100 μm. Data are representative of five independent mice per group. Statistical analysis was performed using unpaired Student’st-tests. Error bars represent s.e.m. of independent experiments. Figure 2: Dnmt1 is indispensable for mammary stem/progenitor cell maintenance. ( a ) Single-cell suspensions from mammary glands of Dnmt1 fl/fl and Dnmt1 Δ/Δ mice were stained with CD24, CD49f and Lin (CD31, CD45 and CD119) antibodies. Representative FACS dot blots showing reduced stem (Lin − CD49f high CD24 + ) and luminal cells (Lin − CD49f low CD24 + ) in Dnmt1 -knockout mice ( n =3–5 mice in each). Bar diagram represents per cent of total stem and luminal cell populations in the respective mammary glands. ( b ) Similarly, single-cell suspensions from mammary glands of Dnmt1 fl/fl and Dnmt1 Δ/Δ mice were stained with CD61, CD49f and Lin antibodies. Representative contour blots show reduced luminal progenitor cells (Lin − CD49f low CD61 + ) in Dnmt1 -knockout mice. Bar diagram represents per cent of total ER + and ER − cell populations in the respective mammary glands. ( c ) Representative images show a decrease in size and number in mammospheres generated with cells from Dnmt1 Δ/Δ mice compared with cells from Dnmt1 fl/fl mice ( n =3–5). Twenty thousand cells per ml were used in each group. Bar diagram represents total number of mammospheres per 20,000 cells. Scale bar, 100 μm. Data are representative of five independent mice per group. Statistical analysis was performed using unpaired Student’s t -tests. Error bars represent s.e.m. of independent experiments. Full size image Dnmt1 expression is high in CSCs DNMT1 is essential for maintaining epidermal progenitor cells by suppressing differentiation [18] and plays a direct role in the self-renewal of HSCs and their commitment to lymphoid lineages [22] . Although HSC self-renewal is abrogated by conditional gene knockout of Dnmt1 , the mature differentiated haematopoietic lineage is unaffected [17] , [23] . Furthermore, cancer cells maintain stem cell-like gene expression programme with differential methylation pattern [24] . However, the expression status of DNMT1 in normal MaSCs and CSCs has not been well studied. Thus, we examined Dnmt1 expression in mammospheres, enriched with stem/progenitor cells, obtained from normal mouse mammary glands, and tumorospheres, enriched with tumour propagating CSCs, obtained from premalignant and tumour tissues of MMTV-Neu mice. We found that CSCs have higher levels of Dnmt1 expression compared with MaSCs, along with higher levels of Id-1 , an inhibitor of differentiation, and lower levels of β-casein , a differentiation marker ( Supplementary Fig. 3a,b ). Dnmt1 deletion suppresses mammary tumorigenesis Several lines of evidence implicate DNA methylation in cancer pathogenesis [25] , [26] , with changes in DNA methylation patterns found to be contributing to oncogenesis by affecting the expression levels of proto-oncogenes and tumour suppressor genes [14] , [27] . DNA hypomethylation promotes increased expression of oncogenes, whereas DNA hypermethylation silences tumour suppressor genes [14] . However, there is no direct evidence that either mechanism is operative in mammary tumorigenesis. To test the relative contribution of Dnmt1 in mammary tumorigenesis, we crossed Dnmt1 Δ/Δ mice with MMTV-Neu-Tg mice, which mimic human LP cell of origin [28] , and C3(1)-SV40-Tg, which mimic human basal triple-negative breast cancer [29] . Over 85% of Dnmt1 -mutant mice were resistant to Neu-Tg- and C3(1)-SV40-Tg-driven mammary tumour and lung metastasis. About 65% of Dnmt1 fl/fl -MMTV-Neu-Tg mice developed mammary tumour at an average age of 290 days, whereas only 12% of Dnmt1 Δ/Δ -MMTV-Neu-Tg mice developed mammary tumour at an average age of 360 days ( Fig. 3a,b ). The tumours developed in Dnmt1 Δ/Δ -MMTV-Neu-Tg mice were smaller in size, less invasive and unable to metastasize to distant organs such as the lungs ( Fig. 3c,d and Supplementary Fig. 3c ). The overall survival rate of Dnmt1 Δ/Δ -MMTV-Neu-Tg mice was significantly high compared with Dnmt1 fl/fl -MMTV-Neu-Tg mice ( Fig. 3e ). Similar results were observed for Dnmt1 Δ/Δ -C3(1)-SV40-Tg mice ( Fig. 3a,b,d–f and Supplementary Fig. 3d,e ). 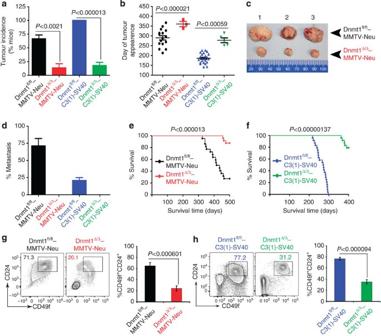Figure 3:Dnmt1deletion suppresses mammary tumorigenesis. Dnmt1Δ/Δmice were crossed with MMTV-Neu-Tg and C3(1)-SV40-Tg mice to generate MMTV-Neu and C3(1)-SV40 transgenic mice in wild-type andDnmt1-null genetic backgrounds. Using these mice, we monitored (a) tumour incidence, (b) age of the animals at tumour onset, (c)tumour size, (d) lung metastasis and (e,f) average survival time. Data are mean±s.e.m. (n=24 mice in each group). (g,h) Representative contour blots show reduced CSC (CD49f+CD24+) in Dnmt1Δ/Δ-MMTV-Neu and Dnmt1Δ/Δ-C3(1)-SV40 mice compared with their respective controls. Bar diagrams represent per cent CSC populations of respective mouse mammary tumours. Data are mean±s.e.m. (n=5 mice in each group). Statistical analysis was performed using unpaired Student’st-tests. Error bars represent s.e.m. of independent experiments. Figure 3: Dnmt1 deletion suppresses mammary tumorigenesis. Dnmt1 Δ/Δ mice were crossed with MMTV-Neu-Tg and C3(1)-SV40-Tg mice to generate MMTV-Neu and C3(1)-SV40 transgenic mice in wild-type and Dnmt1 -null genetic backgrounds. Using these mice, we monitored ( a ) tumour incidence, ( b ) age of the animals at tumour onset, ( c) tumour size, ( d ) lung metastasis and ( e , f ) average survival time. Data are mean±s.e.m. ( n =24 mice in each group). ( g , h ) Representative contour blots show reduced CSC (CD49f + CD24 + ) in Dnmt1 Δ/Δ -MMTV-Neu and Dnmt1 Δ/Δ -C3(1)-SV40 mice compared with their respective controls. Bar diagrams represent per cent CSC populations of respective mouse mammary tumours. Data are mean±s.e.m. ( n =5 mice in each group). Statistical analysis was performed using unpaired Student’s t -tests. Error bars represent s.e.m. of independent experiments. Full size image To test whether the reduced tumour incidence observed in Dnmt1 -knockout mice is simply due to lower number of epithelial cells that are subjected to transformation, we prepared mammosphere from premalignant mammary glands obtained from Dnmt1 fl/fl -MMTV-Neu-Tg and Dnmt1 Δ/Δ -MMTV-Neu-Tg mice, dissociated mammosphere into single-cell suspension and injected the same number (1 × 10 4 ) of single-cell suspension into NOD/SCID mice. Dnmt1 knockout significantly reduced tumour incidence, tumour size and tumorosphere-forming capability ( Supplementary Fig. 3f–h ). These data indicate that delayed tumorigenesis in Dnmt1 knockout is not due to lower number of epithelial cells subject to transformation. Next, we analysed CSC population in tumour tissues of wild-type and Dnmt1 -knockout MMTV-Neu and C3(1)-SV40-Tg mice, using CD24 and CD49f as a CSC marker [30] . Dnmt1 deletion significantly limits the CSC-enriched cell fraction ( Fig. 3g,h ), which is consistent with Dnmt1 activity required for proper renewal of leukemia stem cell [22] . Together, these results suggest that Dnmt1 plays a key role in regulation of CSC self-renewal in mammary epithelium, and that functional deletion of this gene protects mice from mammary tumorigenesis by blocking CSC formation. Inhibition of DNMT activity suppresses mammary tumorigenesis To test whether pharmacological inhibition of DNMTs will block spontaneous mouse mammary tumorigenesis by inhibiting CSC formation, we implanted a sustained slow-releasing DNMT inhibitor 5-azacytidine (5-AzaC) into 12-week-old MMTV-Neu-Tg mice. We also tested the efficacy of histone deacetylase (HDAC) inhibitor butyrate (But) along with 5-AzaC. After confirming reduced DNMT and HDAC activities in cells treated with 5-AzaC and But, respectively ( Fig. 4a,b ), we inspected their tumorosphere-forming capabilities. 5-AzaC implantation alone significantly reduced tumorosphere formation, mammary tumorigenicity and metastasis, and accompanied increased overall survival ( Fig. 4c–f ). The combination of DNMT and HDAC inhibitors greatly enhanced the effect ( Fig. 4g ). As expected, 5-AzaC implantation significantly reduced CSC formation. Interestingly, analysis of CSCs in mice that had not developed tumours in the presence of 5-AzaC and/or But showed three distinct cell populations, stem (CD49f high CD24 + ), luminal (CD49f low CD24 + ) and stromal (CD49f − CD24 − ) cells, instead of a single CSC population (CD49f + CD24 + ) observed for tumour tissues of untreated control mice ( Fig. 4h , top panels). A few animals that were treated with 5-AzaC and/or But developed tumours and these tumours had relatively more CSCs (CD49f + CD24 + ) compared with untreated controls ( Fig. 4h , bottom panels), suggesting that tumour cells that are resistant to 5-AzaC and But might undergo other undefined epigenetic changes that could play a role in CSC regulation. 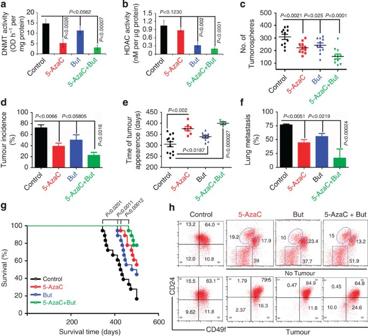Figure 4: Inhibition of DNMT activity suppresses mammary tumorigenesis. (a) DNMT activity was measured in the nuclear extracts prepared from the mammary tumour tissues of untreated control, 5-AzaC, But and the combination (5-AzaC+But). (b) Histone deacetylases activity (HDAC) was measured from the nuclear extract of mammary tumour tissues of untreated control, 5-AzaC, But and the combination (5-AzaC+But). Data represent mean±s.d. of six mice in each group. (c) Tumorospheres number in untreated control, 5-AzaC, But and the combination (5-AzaC+But). Data represent mean±s.d. of three independent experiments. (d–g) Prophylactic treatment of 5-AzaC, But and combination (5-AzaC+But) in MMTV-Neu-Tg mice reduced tumour incidence and delayed tumour growth and lung metastasis with increased overall survival. Data represent mean±s.d. ofn=18 mice per group. (h) Representative FACS dot plot for the untreated control, 5-azaC, But and combination (5-AzaC+But) in MMTV-Neu-Tg mice. Top rows represent the mammary tissues with no visible tumour on treatment with 5-AzaC, But and combination (5-AzaC+But) in MMTV-Neu-Tg mice. Bottom rows represent visible tumours tissues on treatment with 5-AzaC, But and combination (5-AzaC+But) in MMTV-Neu-Tg mice. Statistical analysis was performed using unpaired Student’st-tests. Figure 4: Inhibition of DNMT activity suppresses mammary tumorigenesis. ( a ) DNMT activity was measured in the nuclear extracts prepared from the mammary tumour tissues of untreated control, 5-AzaC, But and the combination (5-AzaC+But). ( b ) Histone deacetylases activity (HDAC) was measured from the nuclear extract of mammary tumour tissues of untreated control, 5-AzaC, But and the combination (5-AzaC+But). Data represent mean±s.d. of six mice in each group. ( c ) Tumorospheres number in untreated control, 5-AzaC, But and the combination (5-AzaC+But). Data represent mean±s.d. of three independent experiments. ( d – g ) Prophylactic treatment of 5-AzaC, But and combination (5-AzaC+But) in MMTV-Neu-Tg mice reduced tumour incidence and delayed tumour growth and lung metastasis with increased overall survival. Data represent mean±s.d. of n =18 mice per group. ( h ) Representative FACS dot plot for the untreated control, 5-azaC, But and combination (5-AzaC+But) in MMTV-Neu-Tg mice. Top rows represent the mammary tissues with no visible tumour on treatment with 5-AzaC, But and combination (5-AzaC+But) in MMTV-Neu-Tg mice. Bottom rows represent visible tumours tissues on treatment with 5-AzaC, But and combination (5-AzaC+But) in MMTV-Neu-Tg mice. Statistical analysis was performed using unpaired Student’s t -tests. Full size image Isl1 is hypermethylated and downregulated in mammary tumours To gain insight into the mechanism by which DNMTs regulate MaSCs and CSCs, we generated genome-scale methylation profiles [31] , [32] using reduced representation bisulfite sequencing of genomic DNA isolated from mammospheres, obtained from normal mouse mammary glands, and tumorospheres, obtained from tumour tissues of MMTV-Neu-Tg mice. We identified 2,341 differentially methylated regions (DMRs) that were either hypermethylated or hypomethylated in tumorospheres compared with mammospheres ( Fig. 5a , Supplementary Fig. 4a–c and Supplementary Data 1 ). A vast majority of DMRs are hypermethylated in tumorospheres ( Supplementary Fig. 4d ), which is consistent with the higher levels of Dnmt1 in tumorospheres ( Supplementary Fig. 3a,b ). Notably, genes associated with hypermethylated CpGs in tumorospheres harbour bivalent histone modifications (activating H3K4me3 and repressive H3K27me3) in MaSCs and LPs ( Supplementary Fig. 4e ), which is consistent with previous reports showing that bivalent genes are often found to be DNA hypermethylated in cancers, and that bivalency may predispose tumour suppressor and pro-differentiation genes for later DNA hypermethylation [33] . 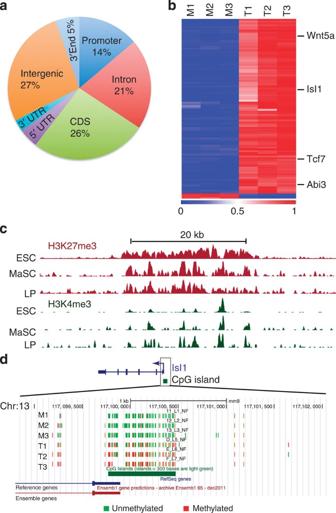Figure 5:Isl1is hypermethylated in mammary tumours. (a) Genome-scale distribution of DMRs identified in mammospheres of normal MaSCs and tumorospheres of tumour-initiating cells prepared from MMTV-Neu-Tg mice (n=3 mice in each). (b) Cluster analysis of top 100 hypermethylated and few hypomethylated genes. (c) Genome browser shot showing chromatin immunoprecipitation sequencing (ChIP-Seq) tracks for H3K27me3 (red) and H3K4me3 (green) levels nearIsl1in embryonic stem cells (ESCs), MaSCs and LPs. (d) UCSC genome browser screenshot showing DNA methylation profile at ISL1 locus in mammospheres and tumorospheres. Red and green colors indicate methylated and unmethylated CpG sites, respectively. Figure 5: Isl1 is hypermethylated in mammary tumours. ( a ) Genome-scale distribution of DMRs identified in mammospheres of normal MaSCs and tumorospheres of tumour-initiating cells prepared from MMTV-Neu-Tg mice ( n =3 mice in each). ( b ) Cluster analysis of top 100 hypermethylated and few hypomethylated genes. ( c ) Genome browser shot showing chromatin immunoprecipitation sequencing (ChIP-Seq) tracks for H3K27me3 (red) and H3K4me3 (green) levels near Isl1 in embryonic stem cells (ESCs), MaSCs and LPs. ( d ) UCSC genome browser screenshot showing DNA methylation profile at ISL1 locus in mammospheres and tumorospheres. Red and green colors indicate methylated and unmethylated CpG sites, respectively. Full size image To identify functional targets of Dnmt1, we focused on 321 genes that are hypermethylated in tumours ( Fig. 5b and Supplementary Data 2 and 3 ). Among the genes are known tumour suppressor genes Wnt5a , Abi3 and Tcf7 , and Isl1 , whose gene product is known to interact with ER [21] ( Fig. 5b and Supplementary Fig. 5a–f ). Consistent with hypermethylation, gene expression analysis revealed a significant downregulation of these genes in CSC-enriched tumorospheres ( Fig. 5b and Supplementary Fig. 5g ). WNT5A is known to be silenced in human breast cancer and loss of WNT5A is associated with early relapse of invasive breast cancer, increased metastasis and poor survival [34] . Similarly, TCF7 is also known to be silenced in breast cancer, with Tcf7-null mice developing spontaneous mammary adenomas [35] . ABI3 expression is frequently lost or reduced in invasive cancer. Ectopic expression of ABI3 inhibits metastasis and cell migration [36] , but ABI3’s mechanism of action is not fully understood. Isl1, a transcription factor, is required for the generation of motor neurons [37] and is a marker for a cardiac progenitor cell lineage that is capable of differentiating into three different cell types of the heart: smooth muscle, cardiomyocytes and endothelial cell types [38] . Isl1 is also known to inhibit ER-driven transcription activation by preventing its dimerization [21] . Given that ERs are overexpressed in ∼ 70% of breast cancer cases, referred to as ‘ER positive’, we sought to investigate the functional link between Isl1 and breast cancer using human and mouse primary breast tumour tissues and human breast cancer cell lines. ISL1 expression negatively correlates with DNMT1 expression Isl1 , bivalent in ESCs and MaSCs ( Fig. 5c ), is hypermethylated in CSC-enriched tumorospheres ( Fig. 5d ). Examination of the TCGA and UCSC Cancer Genomics Database reveal that ISL1 is hypermethylated in a majority of breast cancer subtypes ( Fig. 6a ). Gene expression data from TCGA Pan-cancer show that ISL1 expression is lost or downregulated in many human cancers, and is negatively correlated with the expression of DNMT s in breast cancer ( Supplementary Fig. 6a,b ). Interestingly, ISL1 inactivation is not a common phenomenon in all human cancers; its expression is elevated in some human cancers including pancreatic and prostate cancers ( Supplementary Fig. 6a ), suggesting that the tumour suppressor function of ISL1 is tissue and context dependent. 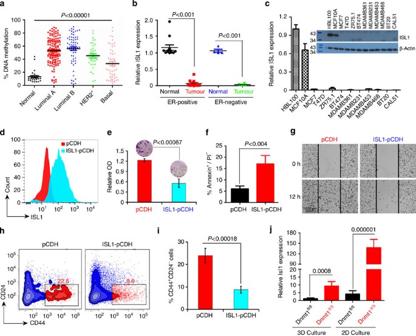Figure 6: ISL1 expression in cancer cells limits CSC population. (a)ISL1promoter was analysed from TCGA human methylation 27K methylation data set at a single CpG site (cg21410991) for differential methylation in luminal A, luminal B, HER2-Neu and basal breast cancer subtypes. (b)ISL1expression in ER-positive (n=12) and negative (n=4) breast tumour and respective normal breast tissues show reduced expression of this gene in both tumour subtypes. (c) ISL1 expression in human non-transformed normal mammary epithelial and human breast cancer cell lines was analysed by quantitative PCR (qPCR) and western blot analysis. (d) Representative FACS data confirming exogenous expression of ISL1 in CAL51 cell line. (e) Representative images of colony-formation assay of CAL51-pCDH and CAL51-ISL1 stable cell lines show that ISL1 expression significantly reduces colony formation. The resulting colonies were stained with Giemsa dye and bound Giemsa dye were dissolved and quantified by spectrophotometer analysis. Data represents mean±s.d. from three independent experiments. (f) Histogram shows that ISL1 expression in CAL51 cells increased apoptosis (Annexin V+/PI−) compared with vector control. Data are mean±s.e.m. of three independent experiments. (g) CAL51-pCDH and CAL51-ISL1 expressing stable cells were subjected toin vitroscratch assay and images were captured using phase-contrast microscope at 12 h after incubation. Scale bar, 200 μm. (h) Representative FACS plot shows decreased CSCs (CD44+CD24−) in ISL1 expressing CAL51 cells. (i) Histogram showing per cent decrease in CSCs after ISL1 expression in CAL51 cells. (j) RelativeISL1expression in wild-type andDNMT1-null mice after three- and two-dimensional culture. (n=3 mice). Statistical analysis was performed using unpaired Student’st-tests. Figure 6: ISL1 expression in cancer cells limits CSC population. ( a ) ISL1 promoter was analysed from TCGA human methylation 27K methylation data set at a single CpG site (cg21410991) for differential methylation in luminal A, luminal B, HER2-Neu and basal breast cancer subtypes. ( b ) ISL1 expression in ER-positive ( n =12) and negative ( n =4) breast tumour and respective normal breast tissues show reduced expression of this gene in both tumour subtypes. ( c ) ISL1 expression in human non-transformed normal mammary epithelial and human breast cancer cell lines was analysed by quantitative PCR (qPCR) and western blot analysis. ( d ) Representative FACS data confirming exogenous expression of ISL1 in CAL51 cell line. ( e ) Representative images of colony-formation assay of CAL51-pCDH and CAL51-ISL1 stable cell lines show that ISL1 expression significantly reduces colony formation. The resulting colonies were stained with Giemsa dye and bound Giemsa dye were dissolved and quantified by spectrophotometer analysis. Data represents mean±s.d. from three independent experiments. ( f ) Histogram shows that ISL1 expression in CAL51 cells increased apoptosis (Annexin V + /PI − ) compared with vector control. Data are mean±s.e.m. of three independent experiments. ( g ) CAL51-pCDH and CAL51-ISL1 expressing stable cells were subjected to in vitro scratch assay and images were captured using phase-contrast microscope at 12 h after incubation. Scale bar, 200 μm. ( h ) Representative FACS plot shows decreased CSCs (CD44 + CD24 − ) in ISL1 expressing CAL51 cells. ( i ) Histogram showing per cent decrease in CSCs after ISL1 expression in CAL51 cells. ( j ) Relative ISL1 expression in wild-type and DNMT1 -null mice after three- and two-dimensional culture. ( n =3 mice). Statistical analysis was performed using unpaired Student’s t -tests. Full size image Using the Gene Set Analysis-Cell line application, we investigated ISL1 messenger RNA expression levels across the breast cancer cell line panel and found that ISL1 is downregulated in a vast majority of breast cancer cell lines ( Supplementary Fig. 6c ). To confirm these data, we analysed ISL1 expression in human primary breast tumour samples and adjacent normal human breast tissue. Although ISL1 transcript level is detectable in normal breast tissues, irrespective of the ER status, ISL1 level is nearly undetectable in tumour samples ( Fig. 6b ). Similarly, irrespective of the ER status, ISL1 expression is low to undetectable in most of the human breast cancer cell lines ( Fig. 6c and Supplementary Fig. 6d ). In addition, examination of Isl1 expression in control and tumour tissues of four different mouse mammary tumour models (MMTV-PyMT-Tg, MMTV-Hras-Tg, MMTV-Neu-Tg and C3(1)-SV40-Tg) revealed relatively low levels of Isl1 in mouse mammary tumour tissues compared with the control tissue ( Supplementary Fig. 6e,f ). Altogether, these results suggested a potential role for ISL1 in suppression of mammary tumorigenesis. ISL1 expression in cancer cells limits CSC population To determine whether the silencing of ISL1 in breast cancer cells is due to DNA hypermethylation, we treated CAL51 and MB231 cells with DNMT inhibitor 5-AzaC and HDAC inhibitor Valproic acid, and found that both inhibitors reactivate ISL1 expression in these cells ( Supplementary Fig. 7a,b ). To study the functional implications of ISL1 in breast cancer, we stably expressed ISL1 in CAL51 cells using a lentiviral vector. After confirming the expression of ISL1 in the stable cell clones ( Fig. 6d and Supplementary Fig. 7c,d ), we investigated the effects of ISL1 expression on cell growth and differentiation, apoptosis and cell migration. Stably expressed ISL1 in cancer cells significantly reduced cell growth and migration, with a significant induction of apoptosis and differentiation ( Fig. 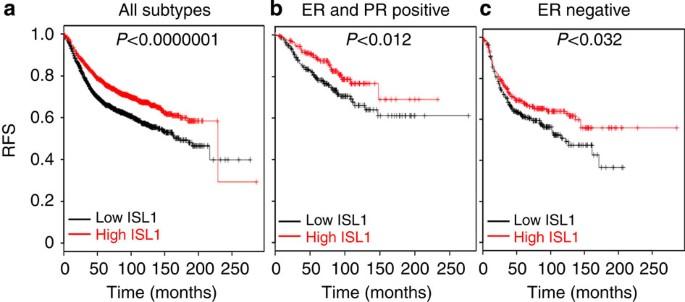Figure 7: Association between ISL1 expression and overall survival. Kaplan–Meier plots of overall survival of breast cancer patients in whole data sets for all breast cancer patients (a), ER positive and progesterone receptor positive patients (b), and ER negative patients (c), stratified by ISL1 expression. Data were obtained from the Kaplan–Meier plotter breast cancer survival analysis database. TheP-value was calculated using a log rank test. 6e–g and Supplementary Fig 7e,f ). To gain insight into ISL1’s role in the regulation of stem cells, we examined the CD44 + CD24 − cell population in CAL51-ISL1 stable cells and found that ISL1 expression significantly reduced CSC population ( Fig. 6h,i and Supplementary Fig 7g ). Together, these data suggest that DNA hypermethylation is one of the causes, if not the cause, for epigenetic silencing of ISL1 in breast cancer cells. Consistent with this conclusion, examination of Isl1 expression in mammosphere derived from the mammary glands of Dnmt1 fl/fl and Dnmt1 Δ/Δ mice revealed significantly elevated levels of Isl1 expression in Dnmt1 -knockout mice ( Fig. 6j ). Association between ISL1 expression and overall survival Finally, to explore the relationship between ISL1 and clinical prognosis, we evaluated the prognostic value of ISL1 in a large clinical microarray database of breast cancer that includes data from 4,142 patients [39] . We found that irrespective of the ER status, low ISL1 expression is associated with poor prognosis and reduced overall survival ( Fig. 7 ), suggesting that ISL1, in addition to its role in the inhibition of oestrogen signalling [21] , may have other roles in blocking mammary tumorigenesis and progression. Figure 7: Association between ISL1 expression and overall survival. Kaplan–Meier plots of overall survival of breast cancer patients in whole data sets for all breast cancer patients ( a ), ER positive and progesterone receptor positive patients ( b ), and ER negative patients ( c ), stratified by ISL1 expression. Data were obtained from the Kaplan–Meier plotter breast cancer survival analysis database. The P -value was calculated using a log rank test. Full size image In this study, we identified a novel role for Dnmt1 in regulating mammary gland development and mammary stem and progenitor cell maintenance. We found that the Dnmt1 -knockout ductal epithelium failed to invade the fat pad and mostly resembled the rudimentary mammary tree that is laid down during embryogenesis, indicating an essential role for Dnmt1 in maintaining the myoepithelial stem cell and LP lineage in the postnatal mammary gland development. Mammary stem and progenitor cell populations are significantly reduced in Dnmt1 -knockout mouse, suggesting a critical role for Dnmt1 in mammary stem and progenitor cell expansion and maintenance. MaSCs proliferate and differentiate during pregnancy and lactation, and interact with stromal cells and extracellular matrix to sustain normal morphogenesis [6] . In the mammary gland, a subpopulation of cells located in the basal layer of terminal end ducts has been implicated as stem cells. We found that deletion of Dnmt1 severely affected TEB development, consistent with reduced number of MaSCs. Together, our data support the conclusion that Dnmt1 is essential for MaSC maintenance. Our findings are in line with recent studies showing a requirement for Dnmt1 is the maintenance of HSCs/progenitor cells [17] , epithelial stem cells [18] and mesenchymal stem cells [18] . Our studies in tumour models provide strong evidence for Dnmt1 playing a critical role in mammary tumour growth and progression. Several lines of evidence implicate DNA methylation in cancer pathogenesis [25] , [26] , with changes in DNA methylation patterns contributing to oncogenesis by affecting the expression levels of proto-oncogenes and tumour suppressor genes [13] , [14] , [27] . DNA hypomethylation has been shown to promote increased expression of many oncogenes, while DNA hypermethylation has been shown to silence tumour suppressor genes [14] . Our studies in human and mouse breast cancer cells show that Dnmt1 deletion decreases tumour formation and metastasis by affecting the self-renewal and proliferation of cancer-initiating cells. Moreover, administration of 5-AzaC and But during premalignant stage efficiently blocked mammary tumorigenesis and reduced tumorosphere-forming potential of CSCs. Together, these results support the conclusion that Dnmt1 is essential for the maintenance of CSCs, which is consistent with a previous study demonstrating an essential role for Dnmt1 in the self-renewal and maintenance of leukemia stem cells [22] . Consistent with the elevated levels of DNMT1 expression in human and mouse cancer cells, a vast majority of DMRs in tumorospheres are hypermethylated compared with mammospheres. Among the hypermethylated genes are known tumour suppressor genes ( Wnt5a , Abi3 and Tcf7 ) and Isl1 , whose gene product is a known inhibitor of ER-driven transcription activation. ISL1 is hypermethylated and downregulated in a majority of breast cancer subtypes, with its expression status negatively correlating with DNMT1 expression. Stable expression of ISL1 or inhibition of DNMT activity successfully limited cellular proliferation and CSC fraction. Together, these data support an essential role for Dnmt1 in tumorigenic phenotype of CSCs and show that inhibition of DNMT activity reverses the abnormal self-renewal properties of CSCs. In summary, our studies provide the first in-vivo evidence that DNMT1 is indispensable for MaSC and CSC maintenance, and that functional inactivation of this gene drastically reduces mammary tumour formation even in the aggressive triple-negative breast cancer subtype. Our results establish ISL1 hypermethylation status as a potential prognostic marker for early breast cancer diagnosis and a role for DNMT1-specific inhibitors in the eradication of CSCs and associated disease recurrence. Animals FVB/NJ (Stock 001800), C57BL/6 (Stock 000664), MMTV-Neu-Tg (Stock 002376), NOD.Cg- Prkdcscid Il2rgtm1Wjl /SzJ (Stock 00557) and C3(1)-SV40-Tg (Stock 013591) mice were obtained from Jackson Laboratories. All these mice were bred and maintained in Georgia Regents University Animal Facility in accordance with the guidelines of the Institutional Animal Care Use Committees. Collection of mammary glands To collect mammary glands from virgin mice, females at ∼ 12 weeks of age without any copulation were used. To collect mammary gland from pregnant mice, females were bred at ∼ 8 weeks of age and copulation was confirmed by plug visualization and males removed post coitum. On 10 and 15 days of pregnancy, mammary glands were collected for analysis. For studies related to lactation, litters were normalized to six pups at birth and mammary glands were collected on 0, 5 and 10 days after delivery. For studies related to involution, pups were removed on day 10 of lactation and mammary glands were collected on day 1, 2, 3, 4 and 8 after the removal of the pups. Generation of Dnmt1-null mice We used Cre/loxP system to conditionally delete Dnmt1 in mammary epithelial cells. Dnmt1 fl/fl mice with loxP sites flanking exons 4 and 5 of the Dnmt1 gene, which were obtained from Mutant Mouse Regional Resource Center at the University of California at Davis (B6.129S4-Dnmt1tm 2Jae /Mmucd, Stock 014114-UCD, Order 146687086), was crossed into MMTV-Cre mice expressing Cre recombinase, which was obtained from Jackson Laboratories (Stock 003553) and generated wild-type (Dnmt1 fl/fl -Cre − or Dnmt1 fl/fl ) and Dnmt1-knockout (Dnmt1 fl/fl -Cre + or Dnmt1 Δ/Δ ) mice. To confirm deletion of Dnmt1, genomic DNA was extracted from the tail snip and the PCR genotype analysis was performed using the following primers: Dnmt1-Fwd: 5′-GGG CCA GTT GTG CTT GG-3′. Dnmt1-Rev: 5′-CTT GGG CCT GGA TCT TGG GGA-3′. To confirm the mammary gland-specific Dnmt1 deletion, RNA and protein samples were prepared from the mammary glands of Dnmt1 fl/fl and Dnmt Δ/Δ mice, and Dnmt1 expression was analysed by quantitative PCR and western blot analyses using specific PCR primers and Dnmt1 antibody. Generation of Dnmt1 −/− -MMTV-Neu-Tg and Dnmt1 −/− -C3(1)-SV40-Tg background Female Dnmt1 Δ/Δ mice were crossed with male MMTV-Neu-Tg mice and the resulting Dnmt1 fl/Δ -MMTV-Neu-Tg mice were intercrossed to generate Dnmt1 fl/fl -MMTV-Neu-Tg and Dnmt1 Δ/Δ -MMTV-Neu-Tg mice. Similarly, female Dnmt1 Δ/Δ mice were crossed with male C3(1)-SV40-Tg mice and the resulting Dnmt1 fl/Δ -C3(1)-SV40-Tg mice were intercrossed to generate Dnmt1 fl/fl -C3(1)-SV40-Tg and Dnmt1 Δ/Δ -C3(1)-SV40-Tg mice. All the littermates generated in this study are in mixed genetic background (Dnmt1 fl/fl mouse was in C57BL/6, MMTV-Cre mouse was in C57BL/6 × 129/Sv, and MMTV-Neu-Tg and C3(1)-SV40-Tg mice were in FVB/N genetic background). We used 8 mice per group and repeated the experiment 3 times, thus giving 24 mice in each group. We monitored time of tumour appearance, tumour size, the number of tumours, and time and per cent of lung metastasis in each mouse. When the mice became morbid due to increased tumour burden and/or lung metastasis, the animals were euthanized and the tumour tissues harvested. If mice did not develop tumour until 500 days of age for MMTV-Neu-Tg and 400 days for C3(1)-SV40-Tg, we considered that these mice are tumour free. Drug treatment For in-vivo studies, we treated 12-week-old female MMTV-Neu-Tg mice with 5-AzaC and sodium But, either alone or in combination, by implanting the respective slow-release pellets (Innovative Research of America) in the back neck region of the animal. We established this experimental procedure recently [40] . These pellets provided a sustained release of 5-AzaC (catalogue number NN-131, 0.5 mg per 90 days) and But (catalogue number NF-125 10 mg per 90 days) for 90 days. Mammary gland single-cell preparation Mammary gland single-cell preparation was carried out as described previously [41] . Briefly, the thoracic and inguinal mammary glands were dissected from virgin and pregnant mice of wild-type, Dnmt1-knockout, MMTV-Neu-Tg and C3(1)-SV40-Tg mice. The tissues were digested for 6–8 h at 37 °C in DMEM/F12 medium supplemented with 10% fetal bovine serum (FBS), 1% Penicillin/Streptomycin (P/S), 750 U ml −1 Collagenase and 250 U ml −1 hyaluronidase. After this step, the organoids were collected by centrifugation and then subjected to trypsin (0.5%) and dispase (5 mg ml −1 ) treatment separately. After centrifugation, ammonium chloride was used for red blood cell lysis. All reagents were obtained from stem cells technology unless stated otherwise. Transplantation assay and whole-mount analysis Animals were anaesthetized using Isoflurane and surgery was performed to inject cells into cleared fat area. Single-cell suspension that prepared from Dnmt1 fl/fl and DNMT1 Δ/Δ mice mammary epithelial cells were implanted into the cleared fat of 3-week-old syngenic female mice. In limiting dilution assays, 1 × 10 2 –1 × 10 5 mammary cells per fat pad were transplanted and the outgrowths were analysed after 6 weeks of transplantation. Mammary repopulating unit frequency was calculated using the online Extreme Limiting Dilution Analysis software. Dissected mammary fat pads were spread onto glass slides, fixed in a 1:3:6 mixture of acetic acid/chloroform/methanol overnight and stained with Carmine in whole mount for 12–18 h. Flow cytometry For isolation of stem/progenitor cells, the following antibodies were used: CD49f and CD24 (Stem Cell Technology and eBioscience, respectively), CD45 and CD31 (BD Bioscience), CD44 and ISL1 (BD Bioscience), and Ter119 and CD61 (eBioscience). Blocking was done for 10 min with rat serum. Cells were stained for 30 min on ice and washed with staining media. Finally, cells were resuspended in staining media containing 7-aminoactinomycin D (1 μg ml −1 ) or DAPI (4′-6-diamidino-2-phenylindole, 1 μg ml −1 ) to stain dead cells. Cells were analysed using a LSR II, Flow-jo and sorted Mo flow cell sorter. For flow cytometric analysis of ISL1 protein expression, CAL51-pCDH and CAL51-ISL1 stable cell lines and HBL-100, MCF10A, MDAMBA231 and MDAMB436 cells were fixed with BD Cytofix fixation buffer and permeablized with BD Phosflow perm buffer. Isl1-PE (BD Bioscience)-conjugated antibody was used. DNMT and HDAC activity assay A commercially available DNMT assay kit (Epigentek, Farmingdale, NY, USA) was used to determine DNMT enzymatic activity as per the manufacturer’s instruction. Similarly, HDAC activity was measured using the commercially available HDAC assay kit (BioVision, CA, USA) as per the manufacturer’s instruction. Nuclear fractions from the mammary glands of control, 5-AzaC, But and the combination of these two (5-AzaC+But) were prepared and used as the source of DNMT and HDAC activities. Cell culture Human immortalized normal mammary epithelial cell lines MCF10A was obtained from ATCC (Manassas, VA) and HBL100 was kindly provided by Dr S. Sukumar (Johns Hopkins University, Baltimore, MD). Human breast cancer cell lines (MCF7, T47D, ZR75.1, BT474, MDAMB361, MDAMB231, MDAMB453, MDAMB468 and BT20) were obtained from ATCC. CAL51 cell line was obtained from DSMZ (Braunschweig, Germany). The MCF10A cells were grown in MEGM complete medium. HBL100 cells were grown in McCoy 5A with 10% FBS. MCF7 and BT20 cells were grown in DMEM medium with 10% FBS. T47D, ZR75.1 and BT474 cells were grown in RPMI 1640 medium with 10% FBS. MDAMB231, MDAMB453 and MDAMB468 cells were grown in Leibovit’s L-15 medium with 10% FBS. CAL51 cell line was grown in DMEM medium with supplemented 20% FBS. All these cell lines have been routinely tested for mycoplasma contamination using the Universal mycoplasma detection kit obtained from ATCC and the last mycoplasma test was performed in February 2013. Mycoplasma-free cell lines were used in all of our experiments. Generation of mammosphere For mammosphere culture, cells were seeded in ultra-low attachment plate in DMEM/F12 medium containing B-27 supplement, basic fibroblast growth factor, recombinant human epidermal growth factor, heparin and P/S [42] . For matrigel culture, cells were seeded on six-well precoated matrigel plates, and after 30 min 10% matrigel with DMEM medium containing supplements were added. For passaging of primary spheres to secondary spheres, trypsin 0.5% along with EDTA was used. Mammospheres were disaggregated with 25-G needle. To make single-cell suspension, dispase (5 mg ml −1 ) was used and cells filtered through a 40-μm filter. Next, cells were centrifuged at 500 g for 5 min and supernatant was discarded. Cells were again resuspended in mammopshere suspension media and cell numbers were counted using the haemocytometer. If single-cell suspension had not been achieved, cells were again disaggregated through a 25-G needle. Cell scratch assay and analysis of apoptosis For cell scratch assay, CAL51-pCDH and CAL51-ISL1 cells were allowed to reach 80% confluence and then serum starved for 24 h. Cells were trypsinized and seeded into Poly lysine-coated six-well plates and allowed to adhere and spread on the substrate completely. Cells were scratched using a 200-μl pipette tip. The culture medium was then changed to standard DMEM with 20% FBS and 1% P/S. Cells were incubated at 37 °C for 12 h and Images were taken. For apoptosis assay, cells were stained with Annexin V and 7-AAD, and analysed by flow cytometer according to the manufacturer’s instruction (BD Bioscience). RNA and DNA isolation and real-time PCR Total RNA was prepared using the pure link RNA Isolation Kit (Invitrogen) or Trizol (Invitrogen). DNA was isolated using the DNeasy Blood and tissue isolation kit, according to manufacturer’s protocol (Qiagen). The quality and concentration of RNA and DNA was determined by Agilent Bioanalyzer/Nano Drop Spectrometer. Isolated and purified total RNA was reverse transcribed by complementary DNA synthesis kit (Invitrogen). Taqman and CT kit was used for real-time expression from the sorted cells. Real-time PCR primers, DNMT1 (Mm01151063_m1) and HPRT (Mm01545399_m1) were designed either from Applied Biosystem site or Harward primer bank site (β-casein, ID1, ID2 and 18s). Clonogenic assays Clonogenic assay was performed as described previously [41] . Briefly, CAL51-pCDH and CAL51-ISL1 cells were seeded in six-well plates at 1 × 10 3 cells per well. Cells were cultured for 2 weeks, changing the medium every 3 days, and then washed with PBS and fixed in 100% methanol for 30 min, followed by staining with KaryoMax Giemsa stain for 1 h. The wells were washed with water and dried overnight at room temperature. Finally, cells were lysed with 1% SDS in 0.2 N NaOH for 5 min and the absorbance of the released dye was measured at 630 nm. Generation of ISL1-pCDH expressing stable cell lines Human ISL1 cDNA, which obtained from Sino Biological Inc., was subcloned into pCDH-CMV-MCS-EF1-Puro vector (System Biosciences, Mountain View, CA) at BamH1/Xba1 site. The resultant plasmid was sequenced to confirm the authenticity of the insert. Recombinant lentivirus was produced by co-transfection into 293FT cells with pCDH and ISL1-pCDH constructs, and three other helper vectors, pLP-1, pLP-2 and pVSVG (Invitrogen), using Lipofectamine 2000 transfection reagent. Lentiviral supernatants were harvested at 72 h post transfection and filtered through a 0.45-μm membrane. CAL51 cells were infected for 48 h with fresh lentivirus expressing either pCDH vector control or ISL1-pCDH construct in medium containing 8 μg ml −1 polybrene, and cultured for an additional 48 h. The cells were selected for puromycin resistance (4 μg ml −1 ) for 1 week and maintained in medium containing 1 μg ml −1 puromycin. The level of ISL1 mRNA expression in CAL51 cells expressing pCDH and ISL1-pCDH constructs were analysed by quantitative PCR. ISL1 protein expression was assessed by FACS and western blot analysis with an antibody specific for ISL1. Western blot analysis Fifty micrograms of the cell lystate was resolved in 8% SDS–PAGE and transferred to nitrocellulose membranes. Membranes were incubated with primary (overnight at 4 °C) and secondary (1 h at room temperature) antibodies; unbound antibodies were removed by washing the membrane with 1 × TBST. Primary antibodies ([DNMT1 (Cell Signaling 1:1,000), ISL1 (BD Bioscience 1:5,000) and β-actin (Sigma 1:25,000)) and respective secondary antibodies (Promega 1:10,000–1:50,0000) were used and visualized using ECL detection system (Thermo Scientific). Uncropped images of the westerns blots are shown in supplementary figures 8 and 9 . Immunofluorescence staining and microscopic imaging Seven-micrometre-thick mammary gland/tumour sections were fixed in 4% paraformaldehyde/methanol at room temperature for 10–15 min, washed three times in PBS and then blocked and permeablized in 10% goat serum, 0.1% Triton X-100 for 1 h. Sections were then incubated in primary antibody overnight at 4 °C, washed in PBS, incubated for 1 h in secondary antibodies, washed in PBST and then mounted in Prolong gold antifade (Invitrogen) solution. Sorted cells were cytospin at 400 × RPM onto Superfrost/Plus slides (Fisher), allowed to air dry, rinsed in PBS and then stored in −80 °C. For surface staining experiments, cells were fixed in 4% PFA (Electron Microscopy Sciences), whereas for nuclear staining experiment (DNMT1) cytospin cells were directly fixed in ethanol. After blocking (1 h in 10% goat serum at room temperature), slides were incubated with primary antibodies (overnight at 4 °C), washed and then hybridized with secondary antibodies (1 h at room temperature), washed and mounted in Prolong Gold. Antibodies used were DNMT1 (Cell Signaling, 1:250), 5meC (N81, Calbiochem) and CD49f (GoH3, R&D, 1:250), Secondary antibodies were purchased from Molecular Probes/Invitrogen: anti-rat/rabbit/mouse Alexa fluor 488 and 568 (1:1,500). All sections were imaged using Laser Scanning confocal microscope. For the quantification of 5 mC-positive cells, pictures were taken in six different locations and manually counted the positive cells. Data are represented as mean±s.e.m. of three independent mouse sections. Bisulfite sequencing and data analyses ‘Reduced representation bisulfite sequencing’ and analysis were performed according to a previously published protocol [43] . Briefly, raw sequences were cleaned using in-house scripts and mapped to the mouse genome release mm9 in the UCSC genome browser using Bowtie after in-silico conversion. The methylation of each CpG was measured to determine the fraction of the number of methylated CpGs. Similarly, we measured the methylation of non-overlapping windows of 200 bp. We filtered out windows that have less than five CpGs. For each window, the methylation difference between normal and tumour groups were calculated by the difference between the average methylation of each group. We used the Student’s t -test for statistical analysis. Multiple testing correction based on FDR generated adjust P -values using a function p adjust in R. DMRs were defined as windows with an adjusted P -value<0.05 and methylation difference >0.25. All DMRs identified were compared using in-house scripts to RefSeq genes, CpG islands and repeats in the UCSC genome browser, and classified into functional categories. The correlation of genome-wide methylation of CpGs common in two samples was calculated by the Pearson’s product–moment coefficient using an R script. Chromatin immunoprecipitation sequencing data analysis Sequence reads were mapped to the mouse genome (mm9) using Bowtie and only those reads that mapped to unique genomic locations with at most two mismatches were retained for further analysis. For visualization on the UCSC Genome Browser and generation of screenshots and read density plots, data were normalized to reads per million and plotted as histograms. DMRs were assigned to the nearest genes (within 50 Kb; RefSeq gene annotations) and read density plots for genes associated with hypermethylated or hypomethylated DMRs in tumorospheres compared with mammospheres were plotted. Published chromatin immunoprecipitation sequencing data sets used for comparative analysis: H3K27me3 in ESCs [44] , H3K4me3 in ESCs (ENCODE and GSE31039), H3K27me3 and H3K4me3 in MaSCs and LPs [7] . Statistical analysis P -value was determined using Student’s t -test with two-tail distribution. Kaplan–Meier analyses ( http://kmplot.com/analysis/ ) were used to assay group differences in tumour-free survival. TCGA data base, UCGC genome, DAVID ( http://david.abcc.ncifcrf.gov ) and GOBO ( http://co.bmc.lu.se/gobo ) were also used to study biological function. Graph pad, sigma plot and excel was used to draw figure. How to cite this article: Pathania, R. et al . DNMT1 is essential for mammary and cancer stem cell maintenance and tumorigenesis. Nat. Commun. 6:6910 doi: 10.1038/ncomms7910 (2015).